Compact genome of the Antarctic midge is likely an adaptation to an extreme environment The midge, Belgica antarctica , is the only insect endemic to Antarctica, and thus it offers a powerful model for probing responses to extreme temperatures, freeze tolerance, dehydration, osmotic stress, ultraviolet radiation and other forms of environmental stress. Here we present the first genome assembly of an extremophile, the first dipteran in the family Chironomidae, and the first Antarctic eukaryote to be sequenced. At 99 megabases, B. antarctica has the smallest insect genome sequenced thus far. Although it has a similar number of genes as other Diptera, the midge genome has very low repeat density and a reduction in intron length. Environmental extremes appear to constrain genome architecture, not gene content. The few transposable elements present are mainly ancient, inactive retroelements. An abundance of genes associated with development, regulation of metabolism and responses to external stimuli may reflect adaptations for surviving in this harsh environment. Loss of the land bridge between South America and the Antarctic Peninsula isolated the southernmost continent ~33 million years ago [1] , yielding a cold, desert environment inhospitable to most forms of terrestrial life. Although the surrounding ocean nurtures an abundance of marine life, and offshore islands offer summer breeding grounds for birds and seals, few animals are found year-round in Antarctica’s terrestrial habitat. Insects, the dominant life form on most continents, are represented by a single endemic Antarctic species, a wingless midge, Belgica antarctica (Diptera: Chironomidae) [2] , [3] , a species first noted by a naturalist aboard the S.Y. Belgica, a Belgian exploratory ship that plied the waters off the Antarctica Peninsula at the end of the 19th century [4] . In its patchy island habitat along the Antarctic Peninsula, B. antarctica is subjected to a range of environmental onslaughts including temperature extremes, periodic desiccation, exposure to both fresh water ice melt and high-salinity sea water, intense ultraviolet exposure, high nitrogen generated from penguin rookeries and elephant seal wallows and high winds [5] , [6] , [7] . The adults, like those of many other species living on wind-swept islands, are apterous (wingless). The larvae ( Fig. 1a ), encased in ice for most of the year, require 2 years to complete their development and then pupate and emerge as adults ( Fig. 1b ) at the beginning of their third austral summer. The apterous adults crawl over surfaces of rocks and other substrates, mate, lay eggs and die within 7–10 days after emergence. 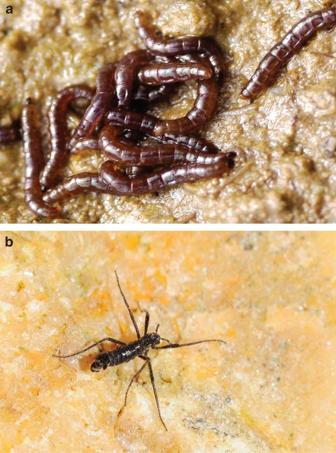Figure 1: Larval and adult stages ofB. antarctica. Fourth (final) instar larvae of the Antarctic midgeB. antarctica(a) and an adult male (b). This is the southernmost insect and the only insect species endemic to Antarctica. Larval length is 6–7 mm, and the adult male is ~3 mm. Photo by Richard E. Lee Jr. Figure 1: Larval and adult stages of B. antarctica. Fourth (final) instar larvae of the Antarctic midge B. antarctica ( a ) and an adult male ( b ). This is the southernmost insect and the only insect species endemic to Antarctica. Larval length is 6–7 mm, and the adult male is ~3 mm. Photo by Richard E. Lee Jr. Full size image Unusual adaptations, including winglessness, freeze tolerance, severe desiccation tolerance and constitutive expression of heat shock proteins [8] , allow this fly to survive in the inhospitable climate of rocky outcrops along the Antarctic Peninsula. The genome of this fly can be expected to offer insights into genomic processes and genome evolution essential to its survival. At the molecular level, select genes that have been examined in B. antarctica include those encoding heat shock proteins [8] , the antioxidant enzymes catalase and superoxide dismutase [7] , a collection of genes that responded to changes in hydration state [9] , [10] and an aquaporin [11] . It is clear from these molecular studies that this species displays some unusual patterns of gene expression. For example, unlike most organisms, the messenger RNAs encoding heat shock proteins, catalase and superoxide dismutase are expressed at high levels all the time, not just in response to a sudden stress. Interestingly, there are also Antarctic fish species that have constitutive expression of heat shock protein 70 (refs 12 , 13 ). The novelty of these responses suggests there are unique genomic adaptations to cope with extreme environments. The genome we present for the extremophile B. antarctica is the first for a dipteran in the family Chironomidae; it consists of 99 megabase pairs assembled using over 100-fold depth coverage of the genome. It is the smallest insect genome discovered thus far. This unusually small genome has low repeat content and general lack of transposable elements (TEs), which are mainly limited to retroelements. The gene content is similar to other Diptera; however, intron length and repeat elements are greatly reduced. Genes that are abundant compared with the related dipteran Anopheles gambiae are associated with development, regulation of metabolism and responses to external stimuli. The genome provides a foundation for studying extremophile biology and insect genome evolution. The genome of B. antarctica is the smallest yet reported for an insect. The estimate of total genome size based on flow cytometry is 1C=99.25±0.4 megabase pairs (Mbp) for the female and 1C=98.4±0.1 Mbp for the male ( Supplementary Methods ; Supplementary Fig. 1 ; Supplementary Table 1 ). On the basis of the raw sequence reads, we estimate the size of the B. antarctica genome to be >89.5 Mbp but <105 Mbp ( Supplementary Fig. 2 ). Previous cytological preparations of polytene chromosomes from salivary glands indicate B. antarctica has three linkage groups (2 n =6) [14] . We used a single larva of B. antarctica of unknown sex from Cormorant Island, near Palmer Station, Antarctica for the reference genome, using Illumina sequencing technology and Velvet de novo [15] for assembly. 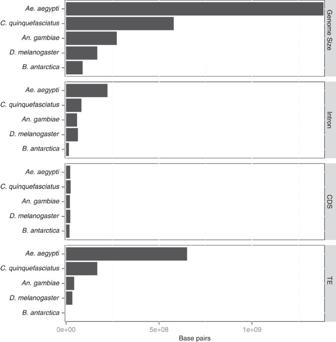Figure 2: Distribution of genome annotations among five Diptera. Each panel is ordered with respect to overall assembled genome size. The four panels represent the total amount of sequence in each annotation: genome size, intron, coding sequence (CDS) and transposable elements (TEs). Several assemblers were compared ( Supplementary Table 2 ). Paired-end reads from RNA-seq data [10] were used to improve the assembly by scaffolding contigs, resulting in 5,064 scaffolds. One Pacific Biosciences RSII SMRTbell library was generated to scaffold the assembly, which added minimal scaffolding owing to the limited amount of DNA in a single individual. The size of the assembled genome was 89.6 Mbp, including ambiguous bases; this represents over 90% of the total genome ( Table 1 ). The assembly consists of 5,003 contigs >300 bp ( Supplementary Fig. 3 ), with an N50 contig length of 98.2 kilobases (kb) and an average coverage of × 177 ( Supplementary Fig. 4 ). A total of 83.89 Mbp (93.7% of the assembled genome) was contained in 1,256 contigs >10 kb. The longest contig assembled was over 622 kb. These multiple lines of evidence as well as the identification of nearly all (97%) core eukaryotic genes suggest a high-quality assembled genome (see also Supplementary Methods ). Table 1 Genome assembly and annotation summary. Full size table The genome of B. antarctica is smaller than even the tiny genomes reported for the body louse (104.7 Mbp) and Strepsiptera (108 Mbp) [16] , [17] . Previously published genome size estimates for three chironomid species, as well as new flow cytometry estimates for three additional members of the family Chironomidae (1C=108–118 Mbp), further suggest that the B. antarctica genome is small even for a chironomid ( Supplementary Methods ; Supplementary Table 1 ). The small genome found in this Antarctic midge does not conform to the coupling frequently reported between low temperatures and large genomes [18] , thus suggesting that alternative evolutionary forces are driving the small size of this genome. The only other Diptera with genomes near 100 Mbp are Colboldia fuscipes (Scatopsidae) and Psycoda cinerea (Psychodidae), cosmopolitan species whose genomes sizes may be constrained by early developmental traits [19] . Amplification, deletion and rearrangements of repeated DNA sequences may account for intraspecific variations in genome size [20] . In B. antarctica the small size of the genome is a function of a paucity of repeats, including a reduction in the number of TEs and the reduced length of introns ( Fig. 2 ). Analysis of the repeat content of the genome assembly revealed that repeat elements comprise only 0.49% of the assembled genome and 10% of the entire genome, assuming that the discrepancy between the assembled genome size and the flow cytometry estimate is due to repeat elements. Most of the repeat elements we identified were found in low-complexity sequences ( Table 2 ; Supplementary Methods ; Supplementary Data 1 ; Supplementary Tables 3–5 ). Using known TE libraries and examining raw reads, we estimate that only 0.016% of the genome failed to assemble due to TE insertions. Furthermore, no species-specific TEs were detected ( Supplementary Methods ). The B. antarctica genome has ~0.12% of the genome as TEs, a small proportion compared with Aedes aegypti (47%) [21] , Anopheles gambiae (16%) [22] , Culex quinquefasciatus (29%) [23] and Drosophila melanogaster (20%) [24] , [25] . In contrast to the above, the body louse Pediculus humanus humanus , similar to B. antarctica , has a small genome (1C=105 Mbp) associated with a low TE proportion (1.03% of genome) [17] . Figure 2: Distribution of genome annotations among five Diptera. Each panel is ordered with respect to overall assembled genome size. The four panels represent the total amount of sequence in each annotation: genome size, intron, coding sequence (CDS) and transposable elements (TEs). Full size image Table 2 Repeat content in B. antarctica . Full size table The TEs found in the B. antarctica genome were of multiple origins. The TEs represent 154 TE families from the three main TE orders (DNA elements, retroelements with long terminal repeat (LTR) and non-LTR retroelements). A total of 513 TE insertion locations were identified in the assembled genome ( Table 2 ). Of those 513 TE insertions, 74 were nested with >1 TE insertion, while the remaining 439 clearly correspond to unique TE insertions. An additional 23 TE insertions were detected as absent from the assembly, as they were located at the flanking regions of the contigs. Most of the unique insertions are from retroelements. The reduced number of TEs in the genome was reflected in ribosomal genes. R1 and R2 non-LTR retroelements are present in nearly all arthropods and have been identified in the ribosomal DNA (rDNA) loci of nearly all arthropod lineages examined to date [26] . However, based on reconstruction of the rDNA region, B. antarctica lacks both R1 and R2 non-LTR retroelements. All lines of evidence suggest that the TE insertions in B. antarctica are of ancient origin. Approximately 19.4% (just under 19 Mbp) of the genome is protein coding in B. antarctica and contains 97% of the core eukaryotic genes ( Supplementary Methods ; Supplementary Tables 6 and 7 ). A large proportion of the genome is coding in comparison with Ae. aegypti (22 Mbp, 1.6% of the genome), An. gambiae (20.7 Mbp, 7.6%), C. quinquefasciatus (24.9 Mbp, 4.3%) and D. melanogaster (22.8 Mbp, 13.6%) ( Fig. 2 ). A total of 13,517 protein-coding genes were annotated, underscoring that loss of gene function is not driving the small genome of B. antarctica. On the basis of a cox1 sequence data, our sample clusters with other samples collected at the same location ( Supplementary Fig. 5 ). Of the 13,517 gene models, 12,914 gene models were supported by at least one RNA-seq read, and 9,011 models were supported by at least 100 RNA-seq reads. Among the annotated genes, 8,575 genes have unique alignments to entries in the SwissProt database, and 10,557 genes have matches in the non-redundant database. Genes are clustered in regions of relatively high GC content (GC content of coding regions is 47%, compared with a 37% GC content for the non-coding, Supplementary Table 8 ). We compared the B. antarctica genome with that of four other dipteran species, three mosquitoes, Ae. aegypti , An. gambiae , C. quinquefasciatus and D. melanogaster , the insect with the most completely annotated genome. Overall, B. antarctica has an intermediate genome GC content but a lower coding GC% than any of the other four Diptera ( Supplementary Table 8 ). Analysis of codon usage suggests that B. antarctica is not unusual compared with the other four dipteran species ( Supplementary Fig. 6 ). Potential clusters of orthologous genes for comparative analyses were determined using annotations from the four dipteran species ( Fig. 3 ). In an orthoMCL [27] comparison between the five species, 4,910 genes were unique to B. antarctica , and 3,582 one-to-one orthologous genes between all five species were identified. Given the lack of TEs in the B. antarctica genome, we interrogated the PIWI-interacting RNA (piRNA) pathway genes ( Supplementary Methods ). The piRNA pathway serves to control transposon activity [28] . We identify several key players in the piRNA pathway that are absent from the B. antarctica genome ( Supplementary Table 9 ). 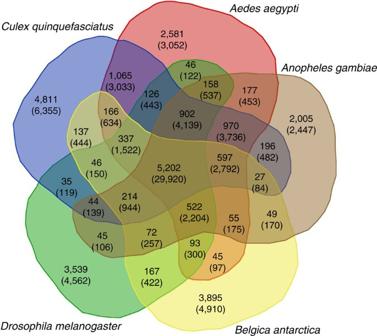Figure 3: Orthologous gene clusters. Venn diagram of orthologous gene clusters amongB. antarctica,An. gambiae,Ae. aegypti,C. quinquefasciatusandD. melanogaster. The numbers in each area indicate the number of orthologous gene clusters in each category, and the numbers in parentheses indicate the total number of genes in each area. The Venn diagram was generated athttp://bioinformatics.psb.ugent.be/webtools/Venn/. Figure 3: Orthologous gene clusters. Venn diagram of orthologous gene clusters among B. antarctica , An. gambiae , Ae. aegypti , C. quinquefasciatus and D. melanogaster . The numbers in each area indicate the number of orthologous gene clusters in each category, and the numbers in parentheses indicate the total number of genes in each area. The Venn diagram was generated at http://bioinformatics.psb.ugent.be/webtools/Venn/ . Full size image Intron size distribution was compared with protein-coding length distribution, calculated for the one-to-one orthologs as well as all genes for each of the five dipteran species ( Supplementary Tables 10–12 ; Supplementary Fig. 7 ). The comparison showed that reduction in intron length also contributed to the reduced size of this genome. While the number of genes is consistent with other Diptera, the relative proportion in different ontologies varies between B. antarctica and An. gambiae . Gene ontology (GO) terms were assigned to the gene models for B. antarctica and the published genes of An. gambiae using Blast2GO [29] ; this yielded 8,856 and 8,653 genes, respectively, with at least one GO term. A comparison of the gene sets using Fisher’s exact test revealed 162 GO terms positively enriched in B. antarctica and 20 terms negatively enriched ( Supplementary Data 2 ). Many of the positively enriched terms fall into two broad categories, ‘development’ (38 terms) and ‘regulation of biological processes’ (50 terms). The effective population size of B. antarctica has been decreasing over the past 10,000 years. Mapping reads onto the assembled genome allowed us to identify 195,860 of the 88,780,579 non-repeat-masked base pairs in the assembled genome as putative heterozygotes; this is an ~0.2% heterozygosity rate, which suggests an average of one heterozygous position for every 450 bp in this single individual (in contrast D. melanogaster has an order of magnitude more heterozygosity at ~2%). The result is similar (~185,000 single-nucleotide polymorphisms (SNPs) in 83.89 Mbp) when the analysis is limited to contigs greater than 10 kb. Using the D. melanogaster single-nucleotide mutation rate of 8.4 × 10 −9 per site per generation (ref. 30 ), we estimate that the time-averaged effective population size of B. antarctica is ~60,000 diploid individuals. We used a pairwise sequentially Markovian coalescent analysis [31] to infer population changes from a single individual to make inferences about population change over time ( Fig. 4 ). Assuming that the mutation rate estimated for B. antarctica is correct, the analysis suggests that the population reached a population size that was maximum just prior to the last glacial maximum, suggesting that the midge populations declined markedly at the glacial maximum but survived in refugia during the period of extensive glaciation. The use of alternate mutation rates would, of course, shift the estimates either higher or lower ( Supplementary Figs 8 and 9 ). Our work is consistent with current hypotheses on Antarctic arthropod dispersal, indicating that most endemic species established well before the last glacial maximum and survived in isolated refugia during glacial periods [32] . Moreover, low levels of genetic diversity suggest a small effective population size, implying that strong selective pressure drove the fixation of adaptive alleles underlying these unique features of the midge genome. 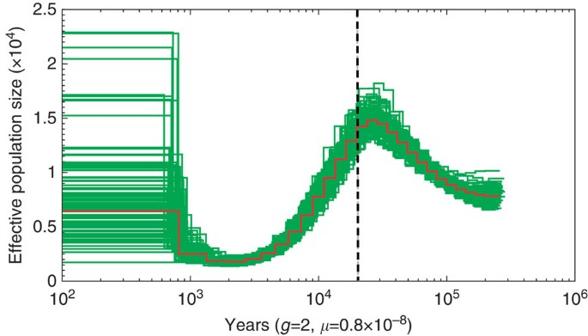Figure 4: Demographic history inferred from a singleB. antarcticagenome. Pairwise sequentially Markovian coalescent (PSMC) analysis for inferred historical population sizes using variant data from the sequenced diploid individual using a mutation rate of 0.84 × 10−8per site per generation. Populations ofB. antarcticareached a maximum size coinciding with the glacial maximum at 20,000 years ago (vertical line on graph). Thexaxis gives time measured by pairwise sequence divergence and theyaxis gives the effective population size measured by the scaled mutation rate. The green lines correspond to PSMC inferences on 100 rounds of bootstrapped sequences, while the red line corresponds to the estimate from the data. Figure 4: Demographic history inferred from a single B. antarctica genome. Pairwise sequentially Markovian coalescent (PSMC) analysis for inferred historical population sizes using variant data from the sequenced diploid individual using a mutation rate of 0.84 × 10 −8 per site per generation. Populations of B. antarctica reached a maximum size coinciding with the glacial maximum at 20,000 years ago (vertical line on graph). The x axis gives time measured by pairwise sequence divergence and the y axis gives the effective population size measured by the scaled mutation rate. The green lines correspond to PSMC inferences on 100 rounds of bootstrapped sequences, while the red line corresponds to the estimate from the data. Full size image The small genome size of B. antarctica is achieved by a reduction in repeats, TEs and intron size, a result similar to that reported for the bladderwort plant ( Utricularia gibba ) [33] and pufferfish ( Tetraodon nigroviridis ) [34] , whose small genomes are also attained by a great reduction in non-genic DNA. Intron size has been correlated to TE number in D. melanogaster [35] , suggesting that in B. antarctica small intron size may be a result of few TEs. There is strong evidence that DNA-mediated transposons (class II) are derived from horizontal gene transfer [36] , [37] ; we hypothesize that horizontal gene transfer events are likely rare in the species-poor Antarctic environment, thus reducing the presence of TEs in Antarctic genomes. While gene content remains largely conserved, the absence of TEs does, however, have a major impact on certain gene classes (for example, the piRNA pathway genes). Moreover, there is evidence that the expression of Hsp90 may be a suppressor of TE movement through either direct interaction with piRNA biogenesis or transposon activation [38] . The constitutive expression of Hsp90 in B. antarctica larvae [8] may also contribute to the lack of active TEs in the genome. Among negatively enriched terms, ‘odourant binding’ suggests a loss of sensory perception in B. antarctica , a feature that may reflect the limited food choices available to the midge in its Antarctic environment, as well as its mating behaviour that does not involve long-distance orientation. By contrast, the mosquito relies extensively on odour reception for the complicated challenges of finding vertebrate hosts and floral nectar sources. It is worth noting that any hypotheses derived from the GO analysis are preliminary, since our comparison was restricted to a single species. The availability of closely related species with well-assembled genomes will facilitate a more in-depth analysis. Notably absent in this genome were genes encoding late-embryogenesis abundant (LEA) proteins; these are critical for surviving extreme dehydration in a close relative, the African sleeping midge, Polypedilum vanderplanki [39] . Dehydration is also a critically important response in larvae of B. antarctica , but in this species other genes, including constitutively expressed heat shock proteins and genes involved in regulation of autophagy, likely contribute to dehydration survival [10] . Use of a single individual for sequencing imposed technological limitations due to the DNA input requirements needed for an assembly. The fresh mass of the fourth instar larvae used in the study was <1.5 mg, and it contained < 1 μg of DNA. To add Pacific Biosciences RSII (PacBio) data, we prepared the sequencing library from DNA extracted from a second individual. The PacBio data yielded only a modest improvement in assembly connectivity due to the low input of genomic DNA. This highlights the need for long-read sequencing technologies that have low input DNA requirements for assemblies of small organisms that cannot be easily reared in the laboratory or readily collected in the field. In recent times, several additional midge species have arrived in the northern perimeter of the Antarctic Peninsula, but these species are also found in Tierra del Fuego, suggesting that they are recent immigrants from South America [2] . B. antarctica has a single congener, B. albipes , a species restricted to one of the sub-Antarctic islands, Isles Crozet. The B. antarctica genome sets the stage for future comparative genomics of Antarctic and Sub-Antarctic species. As the first polar insect and first freeze-tolerant insect to be sequenced, B. antarctica offers a unique opportunity to probe the genome architecture of an extremophile. Lynch [40] argues that small species-effective size should lead to genome expansion, presumably due to a reduction in efficacy of purifying selection. However, this is the opposite of what we observe. Among the genome’s conspicuous features, in fact, is its small size that is attained without reducing the number of protein-coding genes. By stripping the genome of repeats and TEs and by reducing the length of introns, the genome has been streamlined to the minimum yet reported for an insect. Our interpretation is, therefore, that the small midge genome is the result of genome adaptation via fixation of strongly selected mutations that overcame the opposing action of genetic drift inherent in small populations. Biological sample The single fourth instar larva used for sequencing was collected near Palmer Station, Antarctica (64°46′S, 64°04′W) in January 2011. It was held in its natural substrate at 2 °C and shipped to the Denlinger home laboratory at The Ohio State University, where it was held at 4 °C, under a daily 16:8 h light:dark regime until it was used for sequencing. A single individual was used to reduce assembly issues introduced by genetic heterozygosity. DNA library preparation and sequencing DNA was extracted using the Qiagen DNeasy Blood and Tissue Kit and sheared using a Covaris E220 (Woburn, MA) (duty cycle 10, intensity 5, cycles/burst 200 and time 180 s) to ~400 base pair (bp). Sheared genomic DNA was gel purified and used as input for Illumina sequencing library prep, with end-repair using the NEBNext end-repair kit (E6050L), and A-tailing with Taq polymerase. Ligation to Illumina paired-end adapters (PE‐102-1003) was done using Ultrapure ligase (L603-HC-L) from Enzymatics, and amplification with iProof (Bio-Rad). Agencourt Ampure XP beads were used for clean-up and size selection at each step. The resulting DNA library was sequenced on a single lane of an Illumina HiSeq2000 at the Stanford Center for Genomics and Personalized Medicine. PacBio library preparation and sequencing Genomic DNA was sheared using a G-Tube (Covaris Inc.) to generate 10-kb fragments. The sheared DNA was converted into a SMRTbell library using the SMRT bell Template Preparation Kit 1.0 (Pacific Biosciences, Menlo Park, CA). SMRTbell library templates were sequenced using standard SMRT sequencing with a P4 DNA polymerase on the Pacific Biosciences (PacBio) RSII system according to the manufacturer’s protocol in the Genomics Core at the Washington State University, Pullman, WA. De novo genome assembly Genome size determinations from flow cytometry were produced following procedures described in Hare and Johnston [41] (see also Supplementary Methods ). The assembly individual was sequenced to over 100-fold coverage using one lane of Illumina HiSeq2000 sequencing technology with a 400-bp insert paired-end sequencing library. Filtered sequence reads were assembled using Velvet de novo [15] . Two iterations of ERANGE [42] were used to scaffold the assembled contigs with RNA-sequencing data from pooled larvae [10] ( Supplementary Methods ). Filtered sequence reads were mapped back to the reference genome using Burrows-Wheeler Aligner (bwa) with default parameters [43] . PacBio scaffolding was accomplished using PBJelly (Jelly 14.1.14 with blasr 1.3.1) [44] . Mapped sequence reads to the assembled genome were also used to estimate the percent PCR duplicates in the sequencing library using Picard MarkDuplicates tool [45] and to estimate coverage using BamTools [46] . To assess assembly quality, RNA-sequencing data from pooled larvae [10] was mapped to the assembled genome using Bowtie with default parameters [47] . Repeat annotation Repeat annotation was accomplished using RepeatMaker [48] and T-lex2 de novo pipeline [49] , [50] . The T-lex2 de novo pipeline uses reads mapped to the reference and identifies read pairs for which only one read is mapped successfully, called one-end anchored (OEA) pairs, as well as reads that are partially mapped, called split reads. To discriminate TE sequences from other insertions or reference repeated sequences, the unmapped reads from OEA pairs and split reads are BLATed against a library of TE sequences. Finally, a clustering step defines the TE insertion breakpoint on the reference sequence (here our assembly). To avoid bias of the TE discovery owing to the quality of the TE library, we launched RepeatMasker and the T-lex2 de novo pipeline using three previously curated TE libraries from: (i) the Drosophila , (ii) the An. gambiae TE libraries and (iii) a dipteran repeat library constructed from the 12 Drosophila genomes and An. gambiae (RepBase version 17.08 09-01-2012, http://www.fruitfly.org/data/p_disrupt/datasets/ASHBURNER/D_mel_transposon_sequence_set.fasta version 9.41) [51] . Species-specific TE reconstruction was attempted with ReAs [52] . The R1 and R2 TE reconstruction attempt was a multi-approach attempt. Known R1 and R2 elements were downloaded from NCBI, and BLAST was used to map B. antarctica raw reads to the available R1 and R2 element sequences. Few reads mapped to the rDNA from other species, and with no significant evidence for rDNA sequence. Moreover, we undertook a targeted reassembly of the rDNA region using rDNA sequence from D. melanogaster and An. gambiae . Raw reads were mapped to the D. melanogaster and An. gambiae 18S and 28S rDNA sequence. All reads were used in a targeted reassembly of the region, which was compared with the reference assembly and an assembly from RNA-seq data obtained from Teets et al. [10] using Trinity de novo [53] . All genomic reads were then mapped to the rDNA region using bwa [43] and visually inspected for evidence of insertions or reads with split-mappings of OEA mappings that would be indicative of TE insertion. Gene annotation Gene annotation was accomplished using the MAKER annotation pipeline [54] to map protein homology data, expressed sequence tag evidence and ab initio gene predictions to the draft genome. Protein homology data were provided by protein databases of D. melanogaster and Ae. aegypti obtained from FlyBase [55] and VectorBase [56] , respectively. To avoid spurious matches to repetitive regions of the genome, RepeatMasker was used to mask low-complexity regions [48] . In addition to the included libraries, a custom repeat library for use with RepeatMasker was created with RepeatModeler, RECON, RepeatScout and TRF [57] . Filtered RNA-sequencing reads from Teets et al. [10] were mapped to the repeat-masked genome with Bowtie and TopHat and putative transcripts were assembled with Cufflinks [58] . The putative transcripts were used in MAKER as expressed sequence tag evidence. An iterative approach with four rounds of training was used with MAKER and the training of the ab initio predictors SNAP [59] and AUGUSTUS [60] . The benefit of the iterative approach is that with each round, the gene models improve and consequently training the ab initio predictors improves. For the first round, SNAP was not used and the included ‘fly’ hidden Markov model was used in AUGUSTUS. In subsequent rounds, gene models predicted in the previous round of MAKER were used to generate hidden Markov models for SNAP and AUGUSTUS. Functional annotation was accomplished with Blast2GO [29] , [61] . Transcripts predicted by MAKER were compared using BLAST with the SwissProt database [62] (E<10 −10 ) and the non-redundant database (E<10 −10 ). Transcripts predicted by MAKER and the top 19 BLAST hits (blastx, NR, e-value <0.0001) were loaded into Blast2GO. GO terms were assigned based on BLAST hits and InterProScan results [63] . The set of core eukaryotic genes in the assembled genome was identified using CEGMA [64] . Nuclear transfer RNA were predicted using tRNAscan-SE 1.3.1 (ref. 65) [65] using options -H and -y and Aragorn 1.2.34 (ref. 66) [66] using options -w -t -i116 -l -d ( Supplementary Data 3 ). Comparative analyses For comparative analyses, we used the first annotated isoforms for each locus from the annotations of An. gambiae (12,669) [22] , [67] , Ae. aegypti (15,996) [21] , C. quinquefasciatus (18,954) [23] and D. melanogaster (13,492) [55] . Clusters of orthologous genes between the five species were identified using the OrthoMCL package [27] . Effective number of codons, for codon usage estimates, was calculated using ENCPrime using the implementation of Nc’ that accounts for background nucleotide composition [68] . Sizes of introns and exons were calculated using in-house scripts. Functional enrichment analysis We conducted GO enrichment analysis to determine whether any functional groups of genes were enriched in B. antarctica relative to An. gambiae . GO annotations for B. antarctica and An. gambiae were obtained via Blast2GO [29] , [61] , and compared with the built-in Fisher’s exact test (false discovery rate<0.05). Polymorphism detection We identified SNPs in the individual used for the genome assembly. Putative SNPs were identified by mapping trimmed sequencing reads back to the assembled genome using bwa [43] . We then applied the Genome Analysis Toolkit [69] to the mapped reads for PCR duplicate removal, base quality score recalibration and indel realignment. SNP discovery as well as genotyping was performed using standard hard filtering parameters [70] . Demography from a single genome We estimated the demographic history of the single individual using the pairwise sequentially Markovian coalescent method [31] . This method uses sequence data mapped to the reference genome from a diploid individual to infer ancestral effective population sizes at time points in the past determined by the rate of lineage coalescence at that time. The pairwise sequentially Markovian coalescent method was run on data mapped to contigs larger than 10 kb, with parameters -d 58 and -D 354 limits for coverage and bootstrap sampling was executed 100 times. Accession codes: Data for the Belgica antarctica genome has been deposited in GenBank/EMBL/DDBJ BioProject database under the accession code PRJNA172148 . Raw sequence data has been deposited in GenBank/EMBL/DDBJ sequence read archive under the accession code SRA057118 . How to cite this article: Kelley, J. L. et al. Compact genome of the Antarctic midge is likely an adaptation to an extreme environment. Nat. Commun. 5:4611 doi: 10.1038/ncomms5611 (2014).